Direct links between the vernalization response and other key traits of cereal crops Transcription of the VERNALIZATION1 gene ( VRN1 ) is induced by prolonged cold (vernalization) to trigger flowering of cereal crops, such as wheat and barley. VRN1 encodes a MADS box transcription factor that promotes flowering by regulating the expression of other genes. Here we use transcriptome sequencing (RNA-seq) and chromatin immunoprecipitation sequencing (ChIP-seq) to identify direct targets of VRN1. Over 500 genomic regions were identified as potential VRN1-binding targets by ChIP-seq. VRN1 binds the promoter of FLOWERING LOCUS T-like 1 , a promoter of flowering in vernalized plants. VRN1 also targets VERNALIZATION2 and ODDSOC2 , repressors of flowering that are downregulated in vernalized plants. RNA-seq identified additional VRN1 targets that might play roles in triggering flowering. Other targets of VRN1 include genes that play central roles in low-temperature-induced freezing tolerance, spike architecture and hormone metabolism. This provides evidence for direct regulatory links between the vernalization response pathway and other important traits in cereal crops. Many plants from temperate regions require prolonged exposure to low temperatures, or vernalization, to flower. Vernalization was originally defined in temperate cereals, such as wheat, barley and rye [1] . In these annual crops, vernalization is required to promote the transition to reproductive development, so that without vernalization plants will grow vegetatively for extended periods producing only leaves. Following vernalization, inflorescence development begins and will then proceed rapidly if plants are exposed to long day lengths, which accelerate flowering [2] . The VERNALIZATION1 gene (VRN1) encodes a MADS box transcription factor that is a central regulator of vernalization-induced flowering in cereals [3] , [4] , [5] , [6] . VRN1 is expressed at low levels before vernalization and this limits the rate of progression towards flowering [3] , [4] , [5] , [6] . Prolonged exposure to low temperatures induces the transcription of VRN1 (refs 3 , 4 , 5 , 6 ). Induction of VRN1 begins rapidly with the onset of cold but the initial expression is low and several weeks at low temperatures are required for VRN1 transcripts to accumulate to a level that will promote rapid flowering [3] , [4] , [5] , [6] , [7] , [8] . After vernalization, VRN1 transcript levels remain elevated in leaves and at the shoot apex [5] , [8] . The expression of VRN1 at the shoot apex is likely to promote inflorescence meristem identity, whereas the expression of VRN1 in leaves is required for the long-day flowering response [8] , [9] , [10] , [11] , [12] . Some alleles of VRN1 are actively expressed without prior cold treatment [3] , [4] , [5] , [6] . These alleles have mutations in the proximal promoter or deletions/insertions in the first intron of VRN1 , regions that appear to be required to maintain low levels of VRN1 transcription before vernalization [5] , [13] . Chromatin in the first intron of VRN1 has histone modifications that are thought to maintain an inactive transcriptional state, potentially explaining the role of the first intron in maintaining repression of VRN1 before winter [14] . Sequences in the first intron might also regulate processing of the VRN1 transcript [15] . Several active alleles of VRN1 with deletions or insertions in the first intron have been identified in barley [16] , [17] , [18] , [19] . These reduce the vernalization requirement to different extents and have been used to breed varieties that flower without vernalization, which are grown where winters are warm or where crops are sown in spring [19] , [20] . In addition to flowering without vernalization, varieties of wheat or barley that carry active alleles of VRN1 typically have reduced freezing tolerance [21] , [22] . Molecular analyses have identified potential downstream regulatory targets of the VRN1 gene. These include VRN2 and VRN3 , which, like VRN1 , influence vernalization requirement [20] . VRN2 is a repressor of flowering that is expressed in long days before vernalization, but is downregulated in vernalized plants or in plants that carry active alleles of VRN1 (refs 9 , 10 , 23 , 24 , 25 ). VRN3 encodes the cereal orthologue of FLOWERING LOCUS T (hereafter referred to as FT1 ) (ref. 26 ). In Arabidopsis , the FLOWERING LOCUS T protein is expressed in leaves in long days and then transported to the shoot apex to accelerate inflorescence development [27] . It seems likely that FT1 has a similar function in cereals [28] . FT1 is expressed at low levels before vernalization, irrespective of day length, but is induced by long days in vernalized plants, or in plants that have active alleles of VRN1 (refs 10 , 26 ). Thus, the expression of VRN1 is a prerequisite for long-day induction of FT1 in cereals. Another regulatory target of VRN1 is a second MADS box transcription factor, ODDSOC2 , which represses flowering but is downregulated by vernalization or in plants that have active alleles of VRN1 (refs 29 , 30 ). In addition, a series of C-REPEAT BINDING FACTOR (CBF) genes, which are induced by low temperatures to increase freezing tolerance [31] , show reduced expression in lines that carry active alleles of VRN1 (refs 32 , 33 ). Whether VRN1 directly regulates any of these potential targets is unclear. Optimal seasonal timing of flowering and grain production is critical to adapt cereals to temperate climates. The timing and duration of inflorescence development also influences key components of yield in cereal crops. For these reasons, VRN1 is a major target for selection in cereal breeding. Understanding how VRN1 functions can provide important insights into crop biology and inform future cereal breeding strategies. In this study, we used chromatin immunoprecipitation followed by deep sequencing (ChIP-seq) to identify sequences bound by the VRN1 protein in barley, a model for temperate cereals and related grasses. This identified genes that act downstream of VRN1 in the vernalization response and also revealed direct connections between VRN1 and pathways that control other key traits. Epitope-tagged VRN1 protein accelerates flowering of barley A transgene construct was designed to express the barley VERNALIZATION1 protein (VRN1) fused to six copies of the haemagglutinin epitope tag (amino acid sequence YPYDVPDYA). The VRN1-HA gene construct was derived from the genomic sequence of VRN1 , is driven by the endogenous promoter and has the 3′ UTR of VRN1 , but lacks most of the large first intron ( Fig. 1a ). This construct was transformed into the cultivar Golden Promise, a spring barley amenable to Agrobacterium transformation. Transgenic barley plants that carry the VRN1-HA construct flowered earlier than either wild-type parent line or sibling null lines, which were descended from the same transformation events but did not inherit the transgene ( Fig. 1b–d and Supplementary Fig. 1 ). The earliest flowering lines expressing the VRN1-HA transgene also had reduced final height and fewer grains per spike, with altered grain morphology ( Fig. 1e–g and Supplementary Fig. 1 ). The epitope-tagged version of the VRN1 protein was detectable by immunoblot analysis using an anti-haemagglutinin monoclonal antibody ( Fig. 2a ). Compared with sibling nulls, plants carrying the VRN1-HA construct also had higher total transcript levels of VRN1 (endogenous gene plus VRN1-HA transgene; Fig. 2b ). 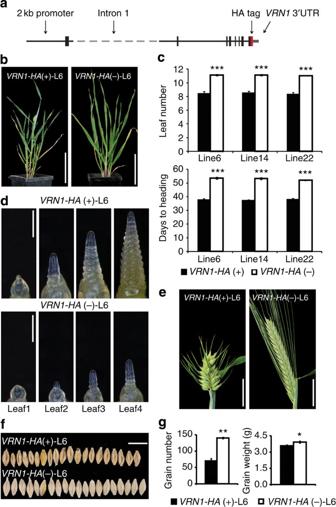Figure 1: A VRN1-HA fusion accelerates the reproductive development in transgenic barley plants. (a) Schematic representation of theVRN1-HAfusion construct, which fuses theVRN1genomic sequence (minus most of first intron) to the coding sequence for six repeats of the haemagglutinin epitope tag (HA). (b) Homozygous plants carrying theVRN1-HAconstruct, from line 6(VRN1-HA(+)-L6) compared with sibling null controls(VRN1-HA(−)−L6) that did not inherit the transgene. Scale bar, 10 cm. (c) The final number of leaves and days to heading of three transgenic lines versus sibling null control plants (n=8). (d) Apex development ofVRN1-HA(+)-L6 andVRN1-HA(−)-L6 from the time of first leaf emergence until the fourth leaf emerged. Scale bar, 500 μm. (e) Spike morphology of plants carrying theVRN1-HAconstruct versus a sibling null. Scale bar, 25 mm. (f) Twenty grains ofVRN1-HA(+)-L6 compared with a sibling null control. Scale bar, 1 cm. (g) Grain number per plant and the weight of 100 grains ofVRN1-HA(+)-L6 plant versus a sibling null control. Stars indicate statistical significance by Student’st-test: *P<0.05, **P<0.01, ***P<0.001. Figure 1: A VRN1-HA fusion accelerates the reproductive development in transgenic barley plants. ( a ) Schematic representation of the VRN1-HA fusion construct, which fuses the VRN1 genomic sequence (minus most of first intron) to the coding sequence for six repeats of the haemagglutinin epitope tag (HA). ( b ) Homozygous plants carrying the VRN1-HA construct, from line 6 (VRN1-HA (+)-L6) compared with sibling null controls (VRN1-HA (−)−L6) that did not inherit the transgene. Scale bar, 10 cm. ( c ) The final number of leaves and days to heading of three transgenic lines versus sibling null control plants ( n =8). ( d ) Apex development of VRN1-HA (+)-L6 and VRN1-HA (−)-L6 from the time of first leaf emergence until the fourth leaf emerged. Scale bar, 500 μm. ( e ) Spike morphology of plants carrying the VRN1-HA construct versus a sibling null. Scale bar, 25 mm. ( f ) Twenty grains of VRN1-HA (+)-L6 compared with a sibling null control. Scale bar, 1 cm. ( g ) Grain number per plant and the weight of 100 grains of VRN1-HA (+)-L6 plant versus a sibling null control. Stars indicate statistical significance by Student’s t -test: * P <0.05, ** P <0.01, *** P <0.001. 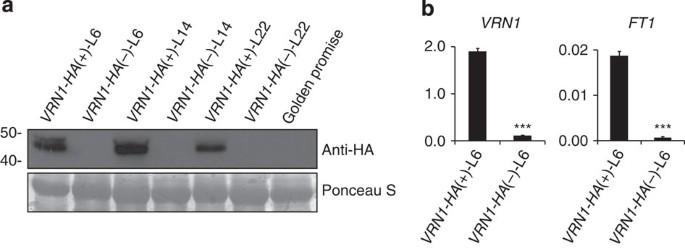Figure 2: Detection of VRN1-HA fusion protein in transgenic barley. (a) Immunoblot detection of the 6xHA-tagged VRN1 protein using a monoclonal anti-HA antibody in plants carrying theVRN1-HAconstruct, from three independent lines (6, 14 and 22) descended from independent transformation events, compared with a sibling null control (line 6) and non-transformed wild-type cv. Golden Promise. Relative positions of 40 and 50 kilodalton markers are indicated. (b) Expression level ofVRN1andFT1, relative toACTIN, inVRN1-HA(+)-L6 compared with a sibling null control. Data are average of three biological replicates, error bar indicates s.e. ***P<0.001 (Student’st-test). Full size image Figure 2: Detection of VRN1-HA fusion protein in transgenic barley. ( a ) Immunoblot detection of the 6xHA-tagged VRN1 protein using a monoclonal anti-HA antibody in plants carrying the VRN1-HA construct, from three independent lines (6, 14 and 22) descended from independent transformation events, compared with a sibling null control (line 6) and non-transformed wild-type cv. Golden Promise. Relative positions of 40 and 50 kilodalton markers are indicated. ( b ) Expression level of VRN1 and FT1 , relative to ACTIN , in VRN1-HA (+)-L6 compared with a sibling null control. Data are average of three biological replicates, error bar indicates s.e. *** P <0.001 (Student’s t -test). Full size image Altered gene expression in lines expressing VRN1-HA To examine how the VRN1-HA construct triggers early flowering, gene expression was assayed by transcriptome sequencing (RNA-seq) at the second leaf stage when the transgenic lines approach inflorescence initiation. DEseq and EdgeR (see Methods) were applied to identify genes that are differentially expressed between a transgenic line (Line 6) and a sibling null control line descended from the same transformation event. These methods detected 678 and 1,283 differentially expressed transcripts, respectively, with 663 genes in common ( Supplementary Data 1 ). Among the overlap between the two methods of analysis were 321 genes that were upregulated and 78 downregulated by twofold or more ( P <0.05, adjusted P value, DEseq or EdgeR). The upregulated genes include a number of genes that potentially promote floral development including VRN1 and VRN1 -like genes ( Barley MADS 3, 8 ), and also four other MADS box genes including a PANICLE ARCHITECTURE2 -like gene. In addition, FT1 and FT2 showed elevated transcript levels in the VRN1-HA positive line. Downregulated genes include a SOC1 -like MADS box gene, a MYB transcription factor, histidine kinase genes and a cytokinin dehydrogenase. Quantitative reverse transcriptase-PCR (qRT–PCR) was used to further verify the expression data for VRN1 and FT1 , and a selection of other differentially expressed genes including Barley MAD3 ( Supplementary Fig. 2 ). Identification of VRN1-binding targets The VRN1-HA protein was used for chromatin immunoprecipitation sequencing (ChIP-seq). Fragments of chromatin bound to the VRN1-HA protein were purified for DNA sequencing on the Illumina HiSeq 2000 sequencing platform. A VRN1-HA transgenic line (Line 6) was compared with a sibling line descended from the same original transgenic plant that did not inherit the transgene (null control). The fold enrichment of sequence reads mapped to the available barley genomic sequence for positive versus sibling null plants was then used to identify sequences bound by the VRN1-HA fusion protein. A total of 514 binding peaks, regions with a bias towards sequence reads in the samples from the positive versus null lines, were identified using 20-fold enrichment as a cutoff value that was chosen on the basis of enrichment of false positives in the null sample ( P <0.05, model-based analysis of ChIP-seq [34] , Supplementary Data 2 ). This dropped to 379 with a 25-fold enrichment limit and 146 with 50-fold enrichment ( Supplementary Data 2 ). Enriched sequence reads were distributed across binding peaks spanning regions from 220 to 1,300 bp in length. Motif analysis of enriched sequences identified two over-represented sequence motifs within the enriched sequences ( Fig. 3a ). One is similar to the CArG box motif (CC[A/T] 6 GG), the typical binding site for MADS box transcription factors. CArG box motifs were found in all the binding peaks, typically located at the centre of peak read distribution ( Fig. 3b ), though there was some sequence variation within the motifs compared with the canonical CArG box sequence ( Fig. 3a ). A second motif, a RY element (CATGCATG), was identified in a subset of 128 of the binding peaks ( Fig. 3a ). 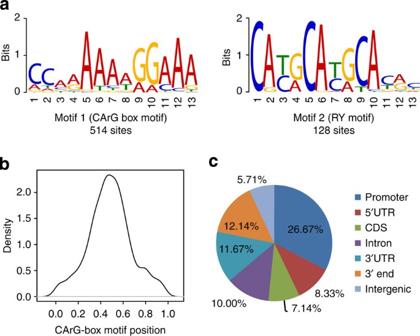Figure 3: Motif analysis of VRN1-HA-binding sequences. (a) Motif analysis of VRN1-HA bound sequences using MEME software. For the distribution of a single motif among the sequences, the parameter was set to zero or one per sequence. (b) The distribution of the CArG box motif within the VRN1-HA-binding regions. (c) Distribution of locations of binding sites relative to target genes. Definitions: promoter is a sequence within 3 kb upstream of TSS (transcription start site); 3′ end is the sequence within 1 kb downstream of TTS (transcription termination site); gene body is dissected into 5′UTR, CDS, intron and 3′UTR; intergenic is anything outside the above regions. Figure 3: Motif analysis of VRN1-HA-binding sequences. ( a ) Motif analysis of VRN1-HA bound sequences using MEME software. For the distribution of a single motif among the sequences, the parameter was set to zero or one per sequence. ( b ) The distribution of the CArG box motif within the VRN1-HA-binding regions. ( c ) Distribution of locations of binding sites relative to target genes. Definitions: promoter is a sequence within 3 kb upstream of TSS (transcription start site); 3′ end is the sequence within 1 kb downstream of TTS (transcription termination site); gene body is dissected into 5′UTR, CDS, intron and 3′UTR; intergenic is anything outside the above regions. Full size image The putative 514 VRN1-binding sites were located on 511 sequenced contigs of the fragmented barley genome assembly, with three having two potential binding sites. A total of 289 of these contigs included predicted genes and associated transcribed sequences. Many (~20%) correspond to transcription factor genes, encoding MYB, B3, Zinc Finger, B-ZIP, MADS box, homeodomain or Leucine Zipper DNA-binding proteins ( Supplementary Data 2 ). Among these were low-temperature-induced C-REPEAT BINDING FACTORS ; CBF2 (Peak 10), CBF4 (Peak 67) and CBF9 (Peak 338; Supplementary Data 2 ). Other potential targets are genes involved in hormone metabolism or regulators of hormone responses. For example, genes encoding enzymes involved in the biosynthesis or breakdown of gibberellins (GA20-oxidase 2, Peak 143), abscisic acid (ABA 8′ Hydroxylase 2, Peak 346) or jasmonic acid (Allene oxide synthase, Peak 269; Supplementary Data 2 ). A number of binding peaks occurred near genes that are likely to regulate reproductive development. One of these was FT1 (Peak 135). Others correspond to CONSTANS -like genes (Peaks 20, 38, 305), SIX ROW SPIKE ( VRS1) (Peak 414), a SUPPRESSOR OF OVEREXPRESSION OF CONSTANS -like MADS box gene (Peak 241) and an ODDSOC2 -like MADS box gene (Peak 154; Supplementary Data 2 ). Mapping the locations of binding sites relative to target genes shows that the locations for putative VRN1-binding sites vary from the promoter to the gene body or the 3′ ends of transcribed sequences ( Figs 3c and 4 ). ChIP-PCR was used to verify the binding of the VRN1-HA protein to a subset of candidate target genes. The majority showed enrichment by both ChIP-PCR and ChIP-seq ( Fig. 5a , Supplementary Fig. 3 ). In addition, ChIP-PCR was used to verify the binding of VRN1-HA to 20 targets that showed a range of different enrichment levels in ChIP-seq ( Supplementary Fig. 3 ). 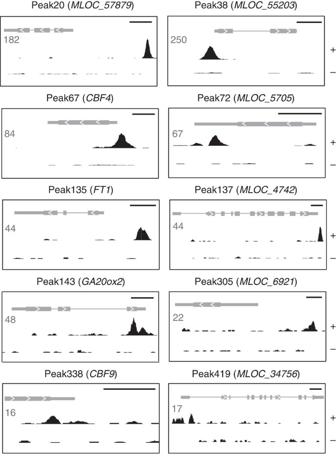Figure 4: Mapping of VRN1-HA-binding sites in putative target genes. Visualization of VRN1-HA binding peaks in 10 selected candidate target genes. Maps were generated using IGV2.3 software. Target gene structures are shown in grey. Thick line indicates exons, medium line indicates untranslated regions and thin lines indicate the location of introns. Overlaid white arrowheads indicate the direction of transcription. The peak height, shown on the left side of each graph, indicates the maximum read number aligning to any region in the target gene. Peak heights for both positive (+) and negative control (−) are shown on the same scale, relative to the maximum number of sequence reads. Black scale bars indicate 500 bp. Figure 4: Mapping of VRN1-HA-binding sites in putative target genes. Visualization of VRN1-HA binding peaks in 10 selected candidate target genes. Maps were generated using IGV2.3 software. Target gene structures are shown in grey. Thick line indicates exons, medium line indicates untranslated regions and thin lines indicate the location of introns. Overlaid white arrowheads indicate the direction of transcription. The peak height, shown on the left side of each graph, indicates the maximum read number aligning to any region in the target gene. Peak heights for both positive (+) and negative control (−) are shown on the same scale, relative to the maximum number of sequence reads. Black scale bars indicate 500 bp. 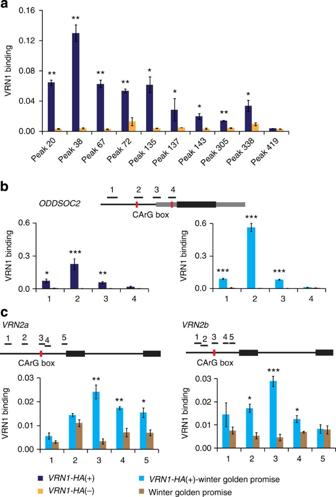Figure 5: Verification of putative VRN1-HA-binding sites by ChIP-PCR. (a) ChIP-PCR was used to verify 10 potential VRN1-HA-binding sites using VRN1-HA line 6 and a sibling null control line. Peak numbers correspond to those inSupplementary Data 2. (b) ChIP-PCR data from multiple sites of the promoter ofODDSOC2in lines carrying the VRN1-HA construct versus sibling null controls. Assay was performed in cv. Golden Promise and in a vernalization-responsive version of the same cultivar, ‘Winter Golden Promise’. Target region is shown in grey. Thick line indicates first exon, medium line indicates transcribed regions and thin lines indicate 5′ upstream sequence. The location of potential MADS box transcription factor-binding sites is indicated in red (CArG box). (c) The binding of VRN1-HA toVRN2aandVRN2b(duplicate genes at theVRN2locus of barley) assayed by ChIP-PCR. VRN1-HA binding was assayed in the Winter Golden Promise background. VRN1 binding indicates relative enrichment, immunoprecipitated DNA versus input chromatin, for three biological repeats. Error bars show s.e. Stars indicate statistical significance by Student’st-test: *P<0.05, **P<0.01, ***P<0.001. Full size image Figure 5: Verification of putative VRN1-HA-binding sites by ChIP-PCR. ( a ) ChIP-PCR was used to verify 10 potential VRN1-HA-binding sites using VRN1-HA line 6 and a sibling null control line. Peak numbers correspond to those in Supplementary Data 2 . ( b ) ChIP-PCR data from multiple sites of the promoter of ODDSOC2 in lines carrying the VRN1-HA construct versus sibling null controls. Assay was performed in cv. Golden Promise and in a vernalization-responsive version of the same cultivar, ‘Winter Golden Promise’. Target region is shown in grey. Thick line indicates first exon, medium line indicates transcribed regions and thin lines indicate 5′ upstream sequence. The location of potential MADS box transcription factor-binding sites is indicated in red (CArG box). ( c ) The binding of VRN1-HA to VRN2a and VRN2b (duplicate genes at the VRN2 locus of barley) assayed by ChIP-PCR. VRN1-HA binding was assayed in the Winter Golden Promise background. VRN1 binding indicates relative enrichment, immunoprecipitated DNA versus input chromatin, for three biological repeats. Error bars show s.e. Stars indicate statistical significance by Student’s t -test: * P <0.05, ** P <0.01, *** P <0.001. Full size image VRN1-binding targets that potentially regulate flowering The potential for binding of VRN1 to influence transcription of nearby genes was examined by comparing ChIP-seq and RNA-seq data at the second leaf stage. A total of 33 differentially expressed transcripts identified by DEseq corresponded to predicted genes located on contigs that have potential VRN1-binding sites. An additional four transcripts identified as differentially expressed by EdgeR were derived from predicted genes located on contigs with VRN1-binding sites. Thus, 37 potential VRN1-binding sites are located near regions that encode transcripts that are differentially expressed at the second leaf stage in lines with elevated VRN1 levels (~13% of annotated transcripts located near VRN1-binding sites). These differentially expressed transcripts include FT1 and also genes encoding zinc finger, B3, zinc finger and MYB transcription factors ( Supplementary Data 3 ). Some targets of VRN1 were strongly upregulated (for example, FT1 ), whereas others were repressed (for example, CBF1 ) suggesting that the binding of VRN1 can activate or repress transcription of target genes ( Supplementary Data 3 ). VRN1-HA binds to the promoters of ODDSOC2 and VRN2 Some potential targets of VRN1 are absent from current barley genome sequence data sets, either due to incomplete genome sequence assembly ( ODDSOC2 ) or due to naturally occurring deletions in the cultivar targeted for sequencing ( VRN2 ). These cannot be identified by the generic ChIP-seq approach used here. Instead qPCR quantification of target DNA in VRN1-HA co-immunoprecipitated chromatin was performed (ChIP-PCR). For ODDSOC2 this was performed using the same Golden Promise transgenic line that was used for ChIP-seq. There was strong enrichment at three sites assayed in the promoter of this gene when chromatin was enriched by immunoprecipitation from the positive versus null control line ( Fig. 5b ). Then, to allow ChIP-PCR analysis of VRN2 , the VRN2 locus was introgressed into Golden Promise, along with a full-length version of VRN1 (requires cold to be actively transcribed) and a functional allele of PHOTOPERIOD1 . As expected, this genotype requires vernalization to flower (hereafter referred to as ‘Winter Golden Promise’) but flowers rapidly when the VRN1-HA construct is present ( Supplementary Fig. 4 ). The binding function of the VRN1-HA fusion in this background was verified by ChIP-PCR using a series of target genes identified by ChIP-seq, plus binding sites from the promoter region of ODDSOC2 . All targets showed strong enrichment in this genotype ( Fig. 5b and Supplementary Fig. 5 ). There was significant enrichment at sites in the promoters for both the duplicate copies of VRN2 , including a region −480 to −360 bp relative to the ATG that is centred around a putative CArG box motif ( Fig. 5c ). Plants that carry the VRN1-HA fusion construct have elevated VRN1 transcript levels and flower earlier than wild-type plants ( Figs 1 and 2 and Supplementary Fig. 1 ). Expression of the transgene is driven by the same promoter as the endogenous gene, so the elevated expression of VRN1 in transgenic plants is likely due to increased overall VRN1 gene copy number (endogenous plus transgene) and possibly the large intron deletion (8.9 kb) that is a feature of the transgene. The early flowering phenotype shows that the VRN1-HA fusion is biochemically active and has the expected biological function. Other phenotypes, such as reduced height and reduced spike length, were observed only in the earliest flowering lines and not in lines with more moderate acceleration of flowering ( Supplementary Fig. 1 ) or in the Winter Golden Promise genotype ( Supplementary Fig. 4 ). Similar phenotypes occur in some non-transgenic early flowering barleys ( Supplementary Fig. 6 ) and are likely a consequence of rapid inflorescence development. Some barley mutants also have similar shortened spikes, which arise from altered rates of inflorescence development. For example, mutants that overexpress HvAPETALA2 (ref. 35 ). Between 146 and 514 direct targets of VRN1 were identified by ChIP-seq, depending on the fold enrichment used as a cutoff value (50 versus 20-fold). Even at the least stringent enrichment limit (20-fold), all the target regions identified contain a potential CArG box motif identified by MEME (Multiple EM for Motif Elicitation [36] ; Supplementary Data 2 ). The false discovery rate values for peaks with more than 20-fold enrichment were generally below 5% ( Supplementary Data 2 ). Thus, 20-fold enrichment was selected as an arbitrary cutoff point for subsequent discussion, although potentially some genuine targets have been omitted. It is important to note that the current genome sequence reference data sets do not represent the entire barley genome [37] , so some targets present in the ChIP-seq data sets will not be identified by the subsequent bioinformatic analysis. The ChIP-seq data set can be realigned to future genomic reference sequences of barley to address this limitation. Binding of VRN1 to putative targets was retested with a second antibody-epitope tag combination using a VRN1::GFP fusion construct [12] , showing that the enrichment of VRN1-binding sites by ChIP is not dependent on the HA-tag/antibody ( Supplementary Figs 3 and 5 ). A key question for this study is which genes are targeted by VRN1 to promote rapid flowering after vernalization? Putative targets of VRN1 identified by ChIP-seq and ChIP-PCR include known regulators of flowering, such as FT1 , VRN2 and ODDSOC2 . These genes are regulated by vernalization and by active alleles of VRN1 , consistent with the idea that these genes are downstream targets of the VRN1 gene (see Introduction). SOC1 -like and CONSTANS -like genes, which regulate the reproductive development of rice [38] , [39] , were also identified as direct targets of VRN1. FT1 was identified as a direct binding target of VRN1 and also shows altered expression during early development in the early flowering VRN1-HA transgenic plants ( Figs 2 and 4 ). Genetic activation of FT1 is sufficient to accelerate the flowering of barley [26] , consistent with the idea that the activation of FT1 (resulting from elevated VRN1 expression) plays a major role in eliciting the early flowering phenotype of VRN1-HA transgenic plants. ODDSOC2 expression did not differ in Golden Promise plants that carry the VRN1-HA transgene versus sibling null lines, despite being a direct target of VRN1 ( Supplementary Fig. 7 ). Golden Promise already carries an active endogenous allele of VRN1 ( HvVRN1-1 ), so ODDSOC2 might be downregulated by default in this genotype. Comparing the expression of ODDSOC2 in a barley that requires vernalization to flower (low VRN1 activity) versus a near-isogenic line that carries a highly active allele of VRN1 ( HvVRN1-7 ; Supplementary Fig. 8 ) shows that this gene has reduced expression when comparisons are made between genotypes with strongly contrasting VRN1 activity ( Supplementary Fig. 9 ), as reported previously [29] . Similarly, VRN2 expression differed in the near-isogenic lines ( Supplementary Fig. 9 ). The finding that VRN1 directly binds to the promoter of FT1 extends current models of the vernalization response of cereals by revealing a direct connection between the vernalization and photoperiod-response pathways ( Fig. 6 ). A requirement for VRN1 to bind to the promoter of FT1 to activate expression of this key flowering regulator can explain why vernalization is a prerequisite for the acceleration of flowering by long days in temperate cereals. The data presented also support the hypothesized direct regulation of VRN2 by VRN1 (refs 9 , 40 ). Similarly, binding of VRN1 to the promoter of ODDSOC2 (and an additional ODDSOC2 -like gene; Peak 154) supports a role for this gene in the vernalization response pathway. 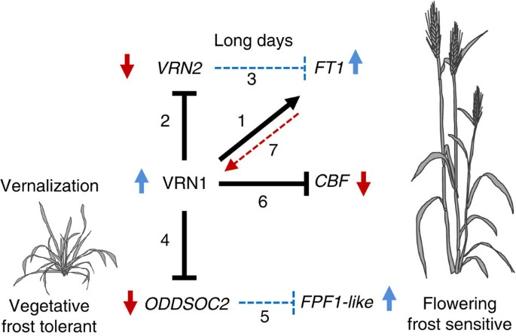Figure 6: A revised model of the molecular network controlling vernalization-induced flowering in cereals. Prolonged exposure to low temperatures (vernalization) induces transcription ofVRN1during winter. Then the VRN1 protein binds to the promoter ofFT1/VRN3(1). This enhances the expression ofFT1in long days. VRN1 also binds to the promoters ofVRN2(2), blocking the expression of this floral repressor and allowing activation ofFT1(3). VRN1 binds to the promoter ofODDSOC2and downregulates this gene (4), allowing the increased expression of other floral promoters (5). Binding of VRN1 to the promoters ofCBFgenes (6) contributes to decreased cold acclimation potential as plants develop towards flowering. Indirect regulation of VRN1 by FT1 can further activate the expression of theVRN1gene in leaves, in long days (7) and can trigger the floral initiation in some genetic backgrounds, but does not play a primary role in vernalization-induced flowering. Direct interactions are indicated by solid black connectors. Regulatory interactions that could be direct or indirect (status unknown) are indicated by thin blue dashed lines. Indirect feedback regulation of VRN1 by FT1 is indicated by a thin red dashed line56. Blue upwards arrows indicate increased expression, red arrows facing downwards indicate decreased expression. Figure 6: A revised model of the molecular network controlling vernalization-induced flowering in cereals. Prolonged exposure to low temperatures (vernalization) induces transcription of VRN1 during winter. Then the VRN1 protein binds to the promoter of FT1/VRN3 (1). This enhances the expression of FT1 in long days. VRN1 also binds to the promoters of VRN2 (2), blocking the expression of this floral repressor and allowing activation of FT1 (3). VRN1 binds to the promoter of ODDSOC2 and downregulates this gene (4), allowing the increased expression of other floral promoters (5). Binding of VRN1 to the promoters of CBF genes (6) contributes to decreased cold acclimation potential as plants develop towards flowering. Indirect regulation of VRN1 by FT1 can further activate the expression of the VRN1 gene in leaves, in long days (7) and can trigger the floral initiation in some genetic backgrounds, but does not play a primary role in vernalization-induced flowering. Direct interactions are indicated by solid black connectors. Regulatory interactions that could be direct or indirect (status unknown) are indicated by thin blue dashed lines. Indirect feedback regulation of VRN1 by FT1 is indicated by a thin red dashed line [56] . Blue upwards arrows indicate increased expression, red arrows facing downwards indicate decreased expression. Full size image More broadly, the direct targets of VRN1 include genes involved in jasmonic acid, abscisic acid and gibberellin biosynthesis or breakdown ( Supplementary Data 2 ). The regulation of hormone levels by VRN1 might influence flowering or other aspects of plant development, such as final height. For example, gibberellins accelerate inflorescence development during the long-day flowering response, downstream of VRN1 (refs 41 , 42 ). VRN1 also binds to the promoters of CBF genes that play critical roles in low-temperature induction of freezing tolerance and to VRS1 ( Supplementary Data 2 ), which regulates spike architecture [43] . Thus, in addition to controlling flowering, VRN1 directly targets genes in pathways that control other key traits such as frost tolerance. The expression analyses presented in this study focussed on early stages of reproductive development, when a subset of direct targets of VRN1 show altered expression in a spring barley transformed with the VRN1-HA construct ( Supplementary Data 3 ). These genes include several transcription factors of unknown function that could potentially play roles in floral development. Other genes that show altered expression during early development but are not bound by the VRN1 protein might be indirectly regulated by increased activity of the VRN1 gene. For example, the expression of Barley MADS3 , an APETALA -like (AP1) MADS box gene, is possibly activated by increased FT1 activity, since FT -like genes are known to activate the expression of AP1 -like MADS box genes that play critical roles during later stages inflorescence development in cereal [44] , [45] . The majority of potential binding targets of VRN1 do not show altered expression at the second leaf stage (ChIP-seq versus RNA-seq data). One potential reason for this is that the fragmented barley genome sequence limits capacity to associate binding sites with potential transcripts. VRN1-binding sites are often present on short contigs (<5 kb) with no predicted genes. Many of these binding sites might nevertheless be located near transcribed regions. A more complete picture of the association of VRN1-binding sites and differentially expressed transcripts will become apparent as the barley reference genome sequence improves. In addition, some targets of VRN1 are likely to show altered expression only under specific conditions. This is known to be the case for CBF genes targeted by VRN1; HvCBF2 , HvCBF4 and HvCBF9 have reduced expression during low-temperature treatment in lines with elevated VRN1 activity but are not expressed in normal glasshouse conditions [33] . A key objective for future studies will be global analyses of gene expression in specific organs and cell types, combined with matching ChIP-seq analysis of VRN1 targets. It is also possible that other factors are required to act with VRN1 to alter the target gene expression. A second promoter motif, the RY element, was identified in a subset of binding targets. This motif is bound by B3 transcription factors, a large family of proteins that regulate many aspects of plant development and also hormone or stress responses [46] . The binding of VRN1 and B3 transcription factors to common promoters could further modify the expression of some genes. Combinatorial action with other transcription factors through discrete binding sites could also explain why VRN1 binding is associated with the repression of some target genes (for example, VRN2 ) but activation of others (for example, FT1 ). In addition to secondary binding motifs in VRN1 target genes, VRN1 is likely to interact with other MADS box transcription factors when binding to CArG motifs, as indicated by yeast two-hybrid assays [47] , [48] . These proteins could modify the impact of VRN1 on target gene expression via cooperative binding to CArG motifs in target genes. In conclusion, the identification of direct and indirect targets of VRN1 provides deeper insights into how this transcription factor regulates the life cycle of cereal crops and influences other key traits. This knowledge of VRN1 targets can be applied to future crop improvement. For example, mutation of VRN1-binding sites can potentially be used to modify the relationship between the vernalization response and other traits such as frost tolerance, spike architecture or plant height. Plant growth conditions Plants were grown in glasshouses at an average temperature of 20°, daily oscillation ± 4°, sine wave. The day length was 16 h (16 light/8 dark), consisting of natural light and artificial day length extension. The production of near-isogenic barley lines has been described previously [7] , as has the production of transgenic barley plants carrying the VRN1-GFP transgene [12] . Expression of the VRN1-HA protein in transgenic barley The 3′ UTR of VRN1 was amplified from a bacterial artificial chromosome (DQ249273, bp 16,923–17,220 relative to VRN1 cv. Strider, AY750993). This fragment (Fragment 1, primers presented in Supplementary Table 2 ) was placed downstream of six copies of the haemagluttinin epitope sequence (6xHA) and the resulting fragment was then fused to a fragment spanning the distal end of the first intron to the penultimate codon in the eighth exon (Fragment 2, bp 12,190 to 16,911 relative to cv. Strider, DQ249273, primers described in Supplementary Table 2 ). Finally, the promoter, first exon, plus a small segment of the first intron of VRN1 (bp 38 to 2,557 relative to cv. Strider) were subcloned upstream of the VRN1-6xHA-UTR segments. Amplification steps were performed with high-fidelity thermostable DNA polymerase (Accuprime Polymerase, Invitrogen). Coding regions were verified by resequencing. Barley plants were transformed with the VRN1-HA transgene using Agrobacterium transformation of excised embryos of the variety ‘Golden Promise’, as described previously [10] . Golden Promise flowers without vernalization (genotype HvVRN1-1, ΔHvVRN2 ) and is photoperiod insensitive. To produce a vernalization-requiring ‘winter’ version of cv. Golden Promise, full-length versions of VRN1 (that is, no intron deletion) and VRN2 (that is, locus present), plus a functional copy of PHOTOPERIOD1 , where introgressed into Golden Promise through three rounds of recurrent crossing with marker assisted selection. The second backcross generation was then crossed to Golden Promise lines carrying the VRN1-HA transgene (three rounds of backcrossing in total) and homozygous plants selected from the BC3F2 generation. Western blot analysis Protein was extracted from barley seedlings (minus roots) at the second leaf stage in homogenization buffer (10% SDS, 10 mM DTT, 20% v/v glycerol, 0.2 M Tris-HCl, 0.2 M PMSF (phenylmethylsulphonyl fluoride) and Protease inhibitor cocktail and then separated by denaturing polyacrylamide electrophoresis (SDS PAGE) and transferred to PVDF transfer membrane (PolyScreen PVDF Hybridization Transfer Membrane, PerkinElmer). VRN1-HA protein was detected using monoclonal anti-HA antibody (H9658, Sigma) in Tris-buffered saline with Tween 20 buffer (20 mM Tris-HCl, 150 mM NaCl and 0.1% v/v Tween 20, pH 7.6) with 0.2% I-block (Tropix, Bedford, MA) at 1/10,000 dilution. Horseradish peroxidase-conjugated goat anti-mouse antibody (PIE31430, Thermo Scientific) was used for secondary detection at 1/100,000 dilution and Supersignal West Dura Substrate was used for signal detection. Raw images of immunoblot results are presented in Supplementary Fig. 10 . ChIP-Seq and ChIP-PCR Chromatin immunoprecipitation was performed as described previously [49] using barley seedlings (minus roots) at the second leaf stage. In brief, barley seedlings were cut into small pieces and crosslinked with 1% formaldehyde for 15 min. Nuclei were isolated and then chromatin was sonicated to shear DNA to a size range of 100–500 bp and immunoprecipitation was performed with monoclonal anti-HA antibody (H9658, Sigma) at a final dilution factor of 1/2,000. Immune complex was collected by protein G Agarose (Millipore 16–266) and DNA was purified by QIAquick PCR Purification kit (Qiagen 28106). Purified DNA samples were used to prepare libraries with the Illumina TruSeq ChIP sample preparation protocol and then sequenced by Illumina Hiseq 2000 with 90 bp single end reads by the Beijing Genomics Institute (BGI). ChIP–Seq data was analysed with Galaxy [50] . Data quality was checked by FastQC and low-quality reads were trimmed. Then the total reads of VRN1-HA (+) and VRN1-HA (−) were mapped to Morex whole-genome shotgun sequence assembly [37] using Bowtie2 with default parameters (total reads and mapping percentage are shown in Supplementary Table 1 ). The mapped reads were applied to Model-based Analysis of ChIP-Seq [34] with default parameters to identify regions enriched in VRN1-HA (+) relative to VRN1-HA (−) sample and visualized by the Integrative Genomics Viewer (IGV) 2.3 (ref. 51 ). A cutoff fold enrichment of 20 was used to finalize the peak list. The sequences of the binding region were extracted and applied to motif analysis using the MEME 4.7.0 (ref. 36 ). ChIP-PCR was performed using quantitative PCR to assay the degree of enrichment of target genomic DNA by comparing immunoprecipitated chromatin fractions to input chromatin. In all cases, ChIP-PCR comparisons were made between lines carrying the VRN1-HA transgene versus sibling null controls (no transgene). Mock immunoprecipitations (no antibody) were also performed as negative controls. Primer sequences are provided in Supplementary Table 2 . Gene expression RNA was extracted using the method of Chang et al . [52] Total RNA (5 μg) was reverse transcribed with Super Script III reverse transcriptase (Invitrogen, www.invitrogen.com ), according to the manufacturer’s instructions. qRT–PCR was performed on a 7900HT Fast Real-Time PCR System (Applied Biosystems, http://www.appliedbiosystems.com ) with SYBR green and Platinum DNA polymerase (Invitrogen). The barley ACTIN gene was used as reference and relative transcript levels of biosynthesis were calculated with the ΔΔ C t method, factoring in primer amplification efficiencies. Primers used are described in Supplementary Table 2 . RNA-seq was performed using three biological replicates of RNA extracted from whole plants (minus roots) at the second leaf stage. RNA was used to generate libraries with the Illumina TruSeq RNA v2 protocol and then sequenced using the Illumina HiSeq platform (100 bp paired end reads) at the Australian Genome Research Facility using standard protocols. The Illumina CASAVA1.8 pipeline was used to generate sequence data. Data quality was checked by FastQC and low-quality reads were trimmed. Sequences were then aligned to the complete CDS contigs from the barley sequencing consortium ( http://www.public.iastate.edu/ ) using Biokanga (version 3.4.2). Differential expression analysis was performed using DEseq [53] (version 1.12.1) and edgeR [54] (version 3.2.4, Robinson 2010), with normalization by model-based scaling normalization or Trimmed Mean of M-values (TMM), respectively. Gene copy number was assayed using the same protocol as qRT–PCR, but with primers targeting the transgene ( Supplementary Table 2 ). The CO2 gene, described previously as a single-copy reference gene [55] , was used for normalization ( Supplementary Table 2 ). How to cite this article: Deng, W. et al . Direct links between the vernalization response and other key traits of cereal crops. Nat. Commun. 6:5882 doi: 10.1038/ncomms6882 (2015). Accession codes: ChIP-seq data has been submitted to the NCBI Sequence Read Archive (SRP041049). RNA-seq data was submitted to the NCBI Sequence Read Archive ( SRP045121 ).